Filopodia-based Wnt transport during vertebrate tissue patterning Paracrine Wnt/β-catenin signalling is important during developmental processes, tissue regeneration and stem cell regulation. Wnt proteins are morphogens, which form concentration gradients across responsive tissues. Little is known about the transport mechanism for these lipid-modified signalling proteins in vertebrates. Here we show that Wnt8a is transported on actin-based filopodia to contact responding cells and activate signalling during neural plate formation in zebrafish. Cdc42/N-Wasp regulates the formation of these Wnt-positive filopodia. Enhanced formation of filopodia increases the effective signalling range of Wnt by facilitating spreading. Consistently, reduction in filopodia leads to a restricted distribution of the ligand and a limited signalling range. Using a simulation, we provide evidence that such a short-range transport system for Wnt has a long-range signalling function. Indeed, we show that a filopodia-based transport system for Wnt8a controls anteroposterior patterning of the neural plate during vertebrate gastrulation. Communication among cells by paracrine signalling is essential for developmental processes, tissue regeneration and stem cell regulation, and its deregulation is also a major cause of diseases such as cancer. The highly conserved family of Wnt proteins contains important regulators for all of the above-mentioned processes [1] , [2] . Wnt proteins are secreted as palmitoylated glycoproteins and can act as morphogens to induce responses in a concentration-dependent manner [3] . The secretion of the Wnt ligand and its presentation at the plasma membrane depends on the function of Evi/Wls, the retromer complex and a functional microtubule network [4] . However, whether Wnt proteins must be secreted from the source cell to fulfil their morphogenetic activity was recently challenged in flies when it was found that a membrane-tethered form of the ligand rescued the Drosophila Wg mutant [5] . Thus, there is still considerable debate regarding the cellular mechanisms that ensure the controlled release and spreading of Wnt morphogens. Several transport mechanisms, such as diffusion with the aid of carrier proteins [6] , [7] or exovesicles, more specifically exosomes [8] , [9] , [10] , have been proposed to play roles in the passage of hydrophobic Wnt molecules through a tissue, most often the Drosophila imaginal wing disc. In those models, however, the source tissue has no control over the direction or range of the signal after release; indeed, these transport mechanisms do not appear to be essential for Wnt gradient formation [9] . Specialized filopodia transmitting signalling proteins between communicating cells would allow a high degree of control of the propagation speed and direction and the concentration of the transmitted ligand. These signalling extensions were first detected in Drosophila and defined as cytonemes [11] , and there is now good correlation between these cellular protrusions and the transport of various signalling molecules, such as the fibroblast growth factor branchless [12] , Notch-Delta ligands [13] , Dpp [14] and Hh proteins [15] . Recently, these thin, actin-positive cytonemes have been identified in the chick limb bud [16] , where they were suggested to establish Shh signalling gradients over several hundreds of micrometres. Other cell protrusions with the potential to transmit signalling factors were defined as tunnelling nanotubes [17] or intracellular bridges [18] . Whether Wnt molecules can be mobilized on cell protrusions is unclear. Porcupine-mediated lipidation of Wnt is important for the secretion [19] , [20] and localization of the ligand to membranes, including membrane protrusions, in zebrafish [21] . However, the mechanism controlling Wnt transport and gradient formation after it is localized to the membrane in a vertebrate tissue, such as the neural plate, is not yet understood. In this study, we report on the presentation of Wnt8a on the tips of specialized Cdc42/N-Wasp-positive, actin-based filopodia on signal-transmitting cells in live zebrafish embryos, in zebrafish PAC2 fibroblasts and HEK293T human embryonic kidney cells. We show the activation of the Wnt/β-catenin signalling pathway at the contact point of the filopodia at the cell body of a neighbouring cell. Furthermore, we show that Cdc42/N-Wasp-dependent short filopodia are required for activation. We hypothesize that such a short-range propagation mechanism is essential for the generation of a morphogenetic field, and we simulate the formation of a long-range gradient based on measured parameters. Finally, we show that such a spreading mechanism is, indeed, crucial during patterning of the central nervous system in vertebrates. Cell extensions carry Wnt protein to neighbouring cells To investigate the spread of Wnt in a living embryo, we focused on Wnt8a as the main Wnt/β-catenin signal during early zebrafish gastrulation and neural plate patterning [22] . Local Wnt sources were generated by mRNA overexpression of a bio-active fluorescently tagged Wnt8a [23] in single clones of 10–15 cells in the neural plate of zebrafish embryos at the 50% epiboly stage (6 h post-fertilization, hpf). To identify Wnt-positive cells, we co-expressed Wnt8a-eGFP together with membrane-tethered fluorescent mCherry-GPI, which illuminates individual epiblast cells within the neural plate in a mosaic manner ( Fig. 1a ). Using this labelling scheme, we observed a dynamic network of thin cellular extensions present on these cells, spanning ~10–50 μm, reflecting several cell diameters, and oriented in many directions from the cell body along the anteroposterior and dorsoventral axes ( Supplementary Movie 1 ) in the living embryo. Intriguingly, we found that fluorescently labelled Wnt8a localized to the distal tips of some cell protrusions ( Fig. 1 , overview Supplementary Fig. 1d ). This subcellular distribution of Wnt8a was also observed in zebrafish PAC2 fibroblasts and HEK293T cells ( Supplementary Figs 2b,4a ). We asked whether overexpression of the tagged Wnt8a protein reflects the localization of the endogenous protein. To localize Wnt8a on a subcellular level, we generated primary cell cultures of several source tissues of zebrafish embryos at the early gastrula stage. Indeed, endogenous Wnt8a protein was detected in cells derived from the marginal zone in intracellular compartments and at the most distal end of cell protrusions ( Supplementary Fig. 1a ). No anti-Wnt8a immunoreactivity could be detected in control cells derived from the animal pole. To further determine whether the localization of Wnt8a is specific, we examined the subcellular distribution of various lipid-modified GFPs. As palmitoylation is important for the membrane association of Wnt8a in zebrafish [21] , we analysed the subcellular distribution of a palmitoylated GFP (Palm-GFP) and a GFP with a general GPI anchor (GPI-GFP). After 6 hpf, all tested membrane-tethered fluorescent proteins showed ubiquitous localization to the membrane, suggesting that lipidation such as palmitoylation does not convey specific localization of Wnt8a to the filopodia tips ( Supplementary Fig. 1b ). In addition, the non-lipid-modified signalling protein Fgf8a-GFP [24] could hardly be detected at the membrane but was observed in the extracellular space ( Supplementary Fig. 1c ). 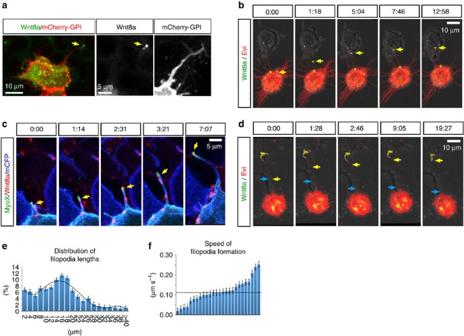Figure 1: Live cell imaging of Wnt8a transport within the zebrafish neural plate and PAC2 fibroblasts. (a) At the 16-cell stage, zebrafish embryos were microinjected in one blastomere with 0.1 ng of mRNA of Wnt8a-GFP and membrane-bound mCherry. Live cell imaging of a 15-μm stack of memCherry expressed in single epiblast cells in a zebrafish embryo at 50% epiboly, highlighting a network of long cytoplasmic extensions. The high magnification pictures of single channels show Wnt8a-GFP localization to the distal tip (arrow,Supplementary Movie 1). (b,c) Series of representative time-lapse images showing (b) PAC2 fish fibroblast transfected with Wnt8a-GFP and Evi-mCherry containing multiple filopodia with Wnt8a present at the distal end (arrow) forming cell–cell contact with a neighbouring PAC2 fibroblast by filopodia (min:s,Supplementary Movie 2). (c) Continuous co-localization of MyoX-GFP with Wnt8a (arrow) during filopodia extension in a zebrafish embryo at 50% epiboly (Supplementary Movie 3). (d) Filopodium pruning process after transfer of Wnt8a-GFP of PAC2 cells (Supplementary Movie 4). After the cuting off, one part of the filopodium is retracted (blue arrows) and the other part shrinks and forms a Wnt8a-positive vesicle at the membrane of the contacted cell (yellow arrow). Scale bars as indicated. Time in min:s. (e) Graph illustrates the distribution of the filopodia lengths of 391 filopodia. Error bars show s.e.m., and a fifth degree polynomial line is displayed. (f) The formation speed of 26 individual filopodia is shown with minimum speed of 0.03 μm s−1up to a maximum of 0.24 μm s−1. Line illustrates mean at 0.11 μm s−1. Figure 1: Live cell imaging of Wnt8a transport within the zebrafish neural plate and PAC2 fibroblasts. ( a ) At the 16-cell stage, zebrafish embryos were microinjected in one blastomere with 0.1 ng of mRNA of Wnt8a-GFP and membrane-bound mCherry. Live cell imaging of a 15-μm stack of memCherry expressed in single epiblast cells in a zebrafish embryo at 50% epiboly, highlighting a network of long cytoplasmic extensions. The high magnification pictures of single channels show Wnt8a-GFP localization to the distal tip (arrow, Supplementary Movie 1 ). ( b , c ) Series of representative time-lapse images showing ( b ) PAC2 fish fibroblast transfected with Wnt8a-GFP and Evi-mCherry containing multiple filopodia with Wnt8a present at the distal end (arrow) forming cell–cell contact with a neighbouring PAC2 fibroblast by filopodia (min:s, Supplementary Movie 2 ). ( c ) Continuous co-localization of MyoX-GFP with Wnt8a (arrow) during filopodia extension in a zebrafish embryo at 50% epiboly ( Supplementary Movie 3 ). ( d ) Filopodium pruning process after transfer of Wnt8a-GFP of PAC2 cells ( Supplementary Movie 4 ). After the cuting off, one part of the filopodium is retracted (blue arrows) and the other part shrinks and forms a Wnt8a-positive vesicle at the membrane of the contacted cell (yellow arrow). Scale bars as indicated. Time in min:s. ( e ) Graph illustrates the distribution of the filopodia lengths of 391 filopodia. Error bars show s.e.m., and a fifth degree polynomial line is displayed. ( f ) The formation speed of 26 individual filopodia is shown with minimum speed of 0.03 μm s −1 up to a maximum of 0.24 μm s −1 . Line illustrates mean at 0.11 μm s −1 . Full size image High-speed in vivo time-lapse analysis of PAC2 fibroblasts revealed that Wnt8-positive protrusions are highly dynamic, including movement and bends in specific subregions as they traverse the extracellular space ( Fig. 1b ). In PAC2 cells, these cell protrusions could be stabilized by connections to neighbouring cells ( Supplementary Movie 2 ). Similarly, in zebrafish embryos, Wnt8a localized predominately to the distal tips of these protrusions during the contact-formation process, as shown by the continuous co-localization of Wnt8a with the filopodia tip marker Myosin X and the formation of stable connections with neighbouring cells ( Fig. 1c , Supplementary Movie 3 ). Approximately 10 min after contact formation, the extensions were shortened, and Wnt8a-positive tips formed extracellular punctae attached to neighbouring cells ( n =12; Fig. 1d , Supplementary Movie 4 ). Zebrafish epiblast cells possessed several cellular protrusions containing Wnt8a. We quantified the lengths of the Wnt-positive cell extensions by 3D scan fragmentation into single epiblast cells, representative surface rendering and the detection of cell protrusions with a maximum diameter of 1.5 μm ( Supplementary Fig. 2a ). We found Wnt-positive filopodia with an average length of 16.6±0.6 μm (mean±s.e.m. ; Fig. 1e ). However, we also detected extensions with a maximum length up to 50 μm in the embryo and up to 70 μm in cultured PAC2 cells ( Supplementary Fig. 2b ). The formation of the extensions displayed an average velocity of 0.11±0.01 μm s −1 ( Fig. 2f ), and this process took <10 min. These observations are consistent with biophysical measurements for actin-based filopodia [25] . 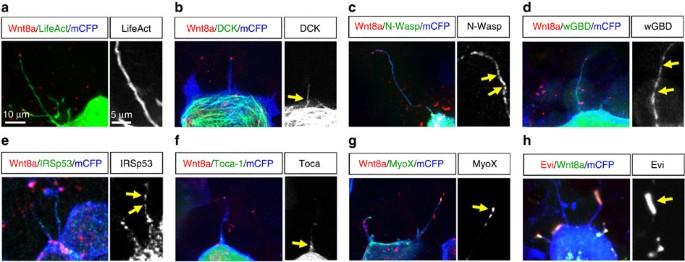Figure 2: Wnt8a is localized on Cdc42/N-Wasp-positive filopodia in epiblast cells of the developing neural plate. (a–h) At the 8–16-cell stage, single blastomeres of zebrafish embryos were microinjected with 0.1 ng of mRNA of indicated constructs to generate focal cell clones at 50% epiboly for confocal microscopy analysis. Live cell imaging of 15-μm stacks of a triple-labelled single epiblast fish cells expressing memCFP, fluorescently tagged Wnt8a and indicated filopodia marker displayed with indicated coloursin vivo. Black and white pictures show higher magnification of Wnt8a-positive filopodia with the indicated markers. Arrows mark localization of indicated proteins at the filopodium base (b,f) in interrupted domains along the filopodium (c–e) and at filopodia tips (g,h). Figure 2: Wnt8a is localized on Cdc42/N-Wasp-positive filopodia in epiblast cells of the developing neural plate. ( a – h ) At the 8–16-cell stage, single blastomeres of zebrafish embryos were microinjected with 0.1 ng of mRNA of indicated constructs to generate focal cell clones at 50% epiboly for confocal microscopy analysis. Live cell imaging of 15-μm stacks of a triple-labelled single epiblast fish cells expressing memCFP, fluorescently tagged Wnt8a and indicated filopodia marker displayed with indicated colours in vivo . Black and white pictures show higher magnification of Wnt8a-positive filopodia with the indicated markers. Arrows mark localization of indicated proteins at the filopodium base ( b , f ) in interrupted domains along the filopodium ( c – e ) and at filopodia tips ( g , h ). Full size image Actin-based filopodia transport Wnt during zebrafish gastrulation Therefore, we asked which cytoskeletal structural proteins are found in the Wnt-positive protrusions and how the formation of these protrusions is regulated. Wnt-positive cytoplasmic extensions were decorated by actin along the entire process, as shown by the highly specific filopodia marker LifeAct ( Fig. 2a , PAC2 cells: Supplementary Fig. 1e ). To visualize tubulin-based structures, the microtubule-associated protein DCK-GFP was used [26] . DCK marked only the proximal base of the protrusions, suggesting that Wnt-positive extensions contain actin bundles but do not contain microtubules ( Fig. 2b ). As a first step in determining the mechanisms regulating the formation of the Wnt8a-containing actin-positive extensions, we focused on the neural Wiskott-Aldrich syndrome protein (N-Wasp) [27] , the small Rho GTPase Cdc42 (ref. 28 ), the Rho family GTPase effector Insulin Receptor tyrosine kinase Substrate p53 (IRSp53) [29] and the transducer of Cdc42-dependent actin assembly 1 (Toca1) [30] . After overexpression, we found that GFP-N-Wasp was present in interrupted domains along Wnt8a-positive protrusions ( Fig. 2c ), a finding that we could replicate when expressing the Cdc42-binding domain of N-Wasp (nGBD-GFP), which labels domains where active Cdc42 is localized [27] ( Fig. 2d ). Next, we analysed the localization of the ubiquitously expressed multidomain scaffold protein IRSp53, which binds active Cdc42 and N-Wasp to promote filopodia formation [31] , [32] and found it in similar microdomains on the filopodium ( Fig. 2e ). The evolutionarily conserved PCH protein Toca1 is one of the earliest localization markers of outgrowing filopodia at the plasma membrane and is thus a core member of the Cdc42/N-Wasp nucleation complex [33] . Toca1-GFP co-localized with Wnt8a-mCherry at the plasma membrane before protrusion formation and was maintained at the proximal part of the filopodium ( Fig. 2f , Supplementary Fig. 1f ). We next examined the localization of a plus-end-directed actin motor, the unconventional Myosin X, which is a member of the filopodia tip complex [34] . MyoX-GFP moved to the distal tips of the filopodia, where it accumulated and co-localized with Wnt8a-mCherry ( Fig. 2g , Supplementary Movie 3 ). Furthermore, the specialized cargo-receptor Evi/Wls binds to Wnts through their palmitate moiety and transfers them to the plasma membrane. Similar to MyoX, Evi-mCherry co-localized with Wnt8a-GFP at these tips ( Fig. 2h ). On the basis of these results, we conclude that Wnt8a is localized to Cdc42/N-Wasp-positive filopodia, along which the protein is transported to the distal tip. Wnt filopodia transduce signalling in the neighbouring cell We wondered whether filopodia act solely as transport vehicles, with Wnt detaching prior to signal activation, or whether they are able to directly activate signalling in the neighbouring cells. Standard in vivo assays for Wnt activity, such as the expression of fluorescent protein driven by multiple repeats of Tcf-responsive elements or the translocation of fluorescently labelled β-catenin into the nucleus, offer low temporal resolution measured in hours and are thus not feasible for showing a quick filopodia-mediated process triggering the activation of a signalling cascade that could operate on the scale of minutes. However, activation of the pathway begins with immediate clustering of the ligand, the transmembrane Frizzled receptors and Lrp5/6 co-receptors at the plasma membrane; these clusters then recruit intracellular Wnt transducers, such as Dishevelled2 (Dvl2) and Axin1, to assemble the so-called Lrp6-signalosome in vitro [35] and in vivo [36] . To address whether Wnt8a-positive filopodia can directly trigger the Wnt cascade in the receiving cells, we expressed fluorescently labelled Wnt8a in a clone of producing cells (P) and expressed fluorescently tagged Lrp6, Dvl2 or Axin1 in an adjacent responding cell clone (R) in gastrulating zebrafish embryos ( Fig. 3a ). We observed co-localization of Wnt8a on filopodia with Lrp6, Dvl2 and Axin1 at the plasma membranes of the receiving cells, whereas Wnt-negative filopodia were unable to cluster these effectors ( Fig. 3b ). This suggests that filopodia-based dispersion directs Wnt8a signal propagation in the gastrulating zebrafish embryo and that these Wnt8a-positive filopodia are able to induce active Lrp6-signalosomes in the neighbouring cells, the first step in Wnt transduction. We could replicate these findings in PAC2 cells in vitro ( Supplementary Fig. 3 ; Supplementary Movie 5 ), suggesting that the mechanism we revealed represents a general mechanism for distributing Wnt proteins rather than a cell- or developmental stage-specific phenomenon. To quantify the signalling capacity of filopodia, Wnt-expressing cells were co-cultivated with cells expressing a Wnt reporter. First, the composition of the actin cortex, including filopodia formation, was perturbed by the chemical inhibition of actin polymerization. Indeed, blockage of actin assembly by Cytochalasin D [37] and Latrunculin B [38] led to a strong reduction in Wnt-positive filopodia in producing cells ( Fig. 3c ). Consistently, treatment with the Cdc42 GTPase inhibitor ML141 [39] resulted in a strong reduction in the number of protrusions formed by PAC2 fibroblasts. 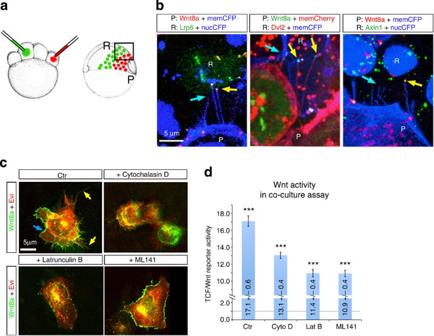Figure 3: Wnt8a-positive filopodia activate signal-responding cells. (a) Schematic presentation of generation of ligand-producing cell clones (P) in close vicinity to responding cell clones (R). At the 16-cell stage, zebrafish embryos were microinjected twice—in one blastomere and the neighbouring blastomere with 0.1 ng of mRNA of each indicated construct. (b) Representative image stacks of live embryos with fluorescently tagged Wnt8a-producing cells (P) that contact the cell body of responding cells (R) expressing Lrp6-GFP; Dvl2-mCherry (for PAC2 cells seeSupplementary Movie 5); and axin1-GFP in a zebrafish embryo at 50% epiboly stage. Yellow arrows show clustering of Lrp6, Dvl2 or Axin1 by Wnt-positive filopodia. Wnt-negative filopodia do not cluster components of the signalosome (blue arrows) (c)In vivoimaging of PAC2 cells transfected with Wnt8a-GFP and Evi-mCherry and treated with indicated inhibitors. Arrows mark Wnt8a-positive filopodia. (d) STF reporter activation of Lrp6 transfected cells co-cultured with Evi-positive, Wnt8a-producing cells after treatment with DMSO (Ctr) and indicated inhibitors. Bars represent fold activation of the STF reporter. Significance level as indicated: ***P<0.005. Figure 3: Wnt8a-positive filopodia activate signal-responding cells. ( a ) Schematic presentation of generation of ligand-producing cell clones (P) in close vicinity to responding cell clones (R). At the 16-cell stage, zebrafish embryos were microinjected twice—in one blastomere and the neighbouring blastomere with 0.1 ng of mRNA of each indicated construct. ( b ) Representative image stacks of live embryos with fluorescently tagged Wnt8a-producing cells (P) that contact the cell body of responding cells (R) expressing Lrp6-GFP; Dvl2-mCherry (for PAC2 cells see Supplementary Movie 5 ); and axin1-GFP in a zebrafish embryo at 50% epiboly stage. Yellow arrows show clustering of Lrp6, Dvl2 or Axin1 by Wnt-positive filopodia. Wnt-negative filopodia do not cluster components of the signalosome (blue arrows) ( c ) In vivo imaging of PAC2 cells transfected with Wnt8a-GFP and Evi-mCherry and treated with indicated inhibitors. Arrows mark Wnt8a-positive filopodia. ( d ) STF reporter activation of Lrp6 transfected cells co-cultured with Evi-positive, Wnt8a-producing cells after treatment with DMSO (Ctr) and indicated inhibitors. Bars represent fold activation of the STF reporter. Significance level as indicated: *** P <0.005. Full size image To investigate the impact of reduced filopodia formation on Wnt signalling, Wnt8a-secreting HEK293T cells were co-cultivated with cells transfected with a Wnt/β-catenin reporter system (SuperTopFlash, STF [40] ). This led to a 17.1-fold increase of STF expression compared with co-cultivation of STF-positive cells with control cells ( Fig. 3d ). On treatment of the co-cultures with the actin polymerization inhibitors Cytochalasin D and Latrunculin B, expression of the STF reporter in the receiving cells was reduced. Cells in which Cdc42 function was blocked with the inhibitor ML141 showed a similar downregulation of STF reporter activation. Cdc42 determines the characteristics of Wnt-positive filopodia To investigate the specific requirement for filopodia formation during secretion, we interfered specifically with Cdc42 activity in Wnt8a-producing cells. We co-transfected Wnt8a-positive HEK293T fibroblasts with Cdc42 wt or the dominant-negative Cdc42 T17N [41] . Furthermore, we blocked Cdc42 activity by overexpressing a mutated form of the Cdc42 effector IRSp53. In the IRSp53 4 K mutant, four lysine residues were mutated to glutamic acid in the actin-binding sites, blocking its actin-bundling function in filopodia [42] . HEK293T fibroblasts transfected with full-length Cdc42 displayed more filopodia with increased length compared with control fibroblasts ( Fig. 4a ). Consistently, HEK293T cells transfected with the dominant-negative Cdc42 T17N or with the mutant form of the Cdc42 effector IRSp53 4 K formed fewer and shorter filopodia. These results were confirmed in fish PAC2 fibroblasts and mouse 3T3 cells ( Supplementary Fig. 4a,b ). Next, to investigate the effect of an increased number of filopodia in Wnt8a-secreting cells on responding cells, we transfected HEK293T cells with Wnt8a and Cdc42 and co-cultured these cells with STF-reporter-positive HEK293T cells. This led to a significant increase in STF expression in co-cultured cells compared with cells transfected with Wnt8a alone ( Fig. 4b ). Consistently, expression of Cdc42 T17N or IRSp53 4 K as well as treatment with the inhibitor Latrunculin B reduced the STF reporter activity in neighbouring cells compared with controls. In summary, these data suggest that Cdc42 facilitates filopodia formation, which in turn enhances non-cell-autonomous Wnt/β-catenin signalling activity. 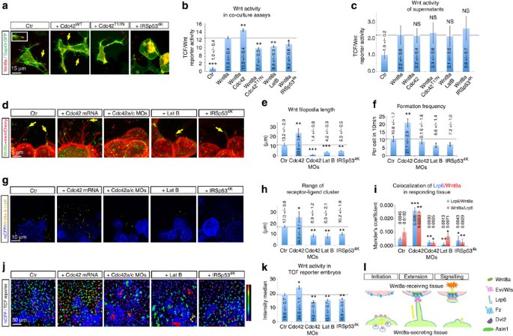Figure 4: Analysis of Cdc42 function during Wnt8a signalling in cell culture and in zebrafish. (a) Transfection of HEK293T cells with Wnt8a showed 14.1±4.1 filopodia with a length of 5.6±1.0 μm. Wnt8a and fulllength Cdc42 transfected fibroblasts displayed 26.8±3.0 filopodia per cell with a length of 7.1±0.5 μm. Cells transfected with Wnt8a and dominant-negative Cdc42T17Nformed 10.0±2.3 filopodia with a length of 4.1±0.2 μm and cells transfected with Wnt8a and IRSp534 Kproduced 12.0±2.9 filopodia with a length of 3.1±0.2 μm (for each experimentsn=15). Inset shows high magnification of Wnt8a-positive filopodium. (b) Cells transfected with Lrp6 and a luciferase-based STF reporter were co-cultivated with cells triple-transfected with indicated constructs. (c) STF activity of supernatants of cells transfected with indicated constructs was analysed (d) Live imaging of cell clones expressing indicated constructs in zebrafish. (e) Filopodia length of clones (n=5) from (d) were quantified and mean of control filopodia is displayed as line. (f) Formation frequency of filopodia per cell in 10 min in five different embryos from (d) were quantified. Mean of formation frequency of control clones is marked. (g) Wnt8a-mCherry+mCFP-positive clones were generated in embryos overexpressing Lrp6-GFP. Representative Lrp6/Wnt8a co-localization and the membrane marker mCFP are displayed with indicated treatments. (h) Quantification of distances of Lrp6/Wnt8a clusters to the source cells from (g). (i) Mander’s co-localization coefficient for Lrp6/Wnt8a was calculated from five clones from (g). Coefficient of 1=full co-localization, 0=random localization. (j) Wnt8+mCFP clones plus indicated constructs were generated in embryos of the Tg(7xTCF-XLa.Siam:mCherry-NLS)ia4zebrafish line. mCherry-positive nuclei were pseudo-coloured according to their mean fluorescent intensity (0=blue, 50=red). (k,h) Quantification of intensity means of nuclei in five different embryos (j). Mean of fluorescence of control nuclei is marked. Significance level as indicated: ***P<0.005, **P<0.01, *P<0.05. (i) Schematic representation of Wnt transport on filopodia. Figure 4: Analysis of Cdc42 function during Wnt8a signalling in cell culture and in zebrafish. ( a ) Transfection of HEK293T cells with Wnt8a showed 14.1±4.1 filopodia with a length of 5.6±1.0 μm. Wnt8a and fulllength Cdc42 transfected fibroblasts displayed 26.8±3.0 filopodia per cell with a length of 7.1±0.5 μm. Cells transfected with Wnt8a and dominant-negative Cdc42 T17N formed 10.0±2.3 filopodia with a length of 4.1±0.2 μm and cells transfected with Wnt8a and IRSp53 4 K produced 12.0±2.9 filopodia with a length of 3.1±0.2 μm (for each experiments n =15). Inset shows high magnification of Wnt8a-positive filopodium. ( b ) Cells transfected with Lrp6 and a luciferase-based STF reporter were co-cultivated with cells triple-transfected with indicated constructs. ( c ) STF activity of supernatants of cells transfected with indicated constructs was analysed ( d ) Live imaging of cell clones expressing indicated constructs in zebrafish. ( e ) Filopodia length of clones ( n =5) from ( d ) were quantified and mean of control filopodia is displayed as line. ( f ) Formation frequency of filopodia per cell in 10 min in five different embryos from ( d ) were quantified. Mean of formation frequency of control clones is marked. ( g ) Wnt8a-mCherry+mCFP-positive clones were generated in embryos overexpressing Lrp6-GFP. Representative Lrp6/Wnt8a co-localization and the membrane marker mCFP are displayed with indicated treatments. ( h ) Quantification of distances of Lrp6/Wnt8a clusters to the source cells from ( g ). ( i ) Mander’s co-localization coefficient for Lrp6/Wnt8a was calculated from five clones from ( g ). Coefficient of 1=full co-localization, 0=random localization. ( j ) Wnt8+mCFP clones plus indicated constructs were generated in embryos of the Tg(7xTCF-XLa.Siam:mCherry-NLS)ia 4 zebrafish line. mCherry-positive nuclei were pseudo-coloured according to their mean fluorescent intensity (0=blue, 50=red). ( k , h ) Quantification of intensity means of nuclei in five different embryos (j). Mean of fluorescence of control nuclei is marked. Significance level as indicated: *** P <0.005, ** P <0.01, * P <0.05. ( i ) Schematic representation of Wnt transport on filopodia. Full size image In addition to the transfer of Wnt by filopodia, Cdc42 may also have the capacity to enhance Wnt spreading by an increasing secretion of Wnt protein into the medium, such as on microvesicles or exosomes. Therefore, we measured the effective signalling capacity of the supernatant of Wnt8a-transfected cells and found that the microfiltered supernatant can activate the reporter expression ( Fig. 4c ). Next, we measured the activity of the supernatants from cells co-transfected with Wnt8a and Cdc42 WT , Cdc42 T17N or IRSp53 4 K and from Wnt8a-producing cells treated with the inhibitor Latrunculin B. We found no significant differences among the Wnt signalling activities of these supernatants, suggesting that Cdc42 mainly regulates Wnt8a on filopodia without increasing secretion to the medium. On the basis of our in vitro experiments, we asked whether Cdc42 has an influence on Wnt8a spreading in the embryo. Therefore, fluorescently tagged Wnt8a and Cdc42 were co-expressed in a clone of neural plate cells, and the length of Wnt-positive cell extensions was determined for five individual clones at 6 hpf ( Fig. 4d ). In this set-up, activation of Cdc42 in the Wnt-producing cells led to an increase in Wnt8a-positive filopodia length and frequency ( Fig. 4e,f ). Furthermore, Cdc42-hyperactive, Wnt-positive filopodia were often branched and displayed Wnt8a at several of their distal tips. To block Cdc42 function in vivo , we performed a Morpholino oligomer-based double-knockdown approach for both Cdc42 homologues, Cdc42a and Cdc42c, which are expressed early in the Wnt-producing cells in zebrafish embryos. Cdc42 double-morphant cells displayed a markedly reduced average length of Wnt8a-positive filopodia ( Fig. 4d,e ). In zebrafish, low concentrations of Latrunculin B have been proven useful to specifically block filopodia formation, leaving the intracellular actin cortex largely intact [43] . Indeed, the filopodia lengths in clones blocked for Cdc42 function were comparable to the length of filopodia after treatment with a low concentration of Latrunculin B. To validate the Morpholino-based knockdown approach, we reduced Cdc42-dependent filopodia formation by expressing IRSp53 4 K . Similar to the Cdc42a/c double-knockdown, we found that the formation of Wnt8a-positive filopodia in zebrafish was decreased on expression of IRSp53 4 K , and their average length was significantly reduced. Although the length of the filopodia was significantly decreased, the frequency of filopodia formation was only slightly affected in the latter treatments ( Fig. 4f ). Next, we quantified the effective signalling ranges of these clones. To this end, the Wnt8a-producing clones were introduced into embryos expressing fluorescently tagged Lrp6 and into live transgenic embryos expressing nuclear mCherry under the control of the β-catenin/TCF responsive elements, Tg(7xTCF-XLa.Siam:mCherry-NLS) ia4 [44] . We measured the range at which Lrp6/Wnt8a clusters could be identified around the source clone ( Fig. 4g,h , Supplementary Fig. 4c ). Formation of ligand-receptor complexes was observed as a halo surrounding the Wnt-positive clone. In addition, the Mander’s co-localization coefficients for Lrp6 with Wnt8a (Mander’s 1) and Wnt8a with Lrp6 (Mander’s 2) were calculated ( Fig. 4i ). When the clones co-expressed Wnt8a and Cdc42, the distance at which the ligand-receptor clusters could be detected was extended, coupled with an increased Mander’s co-localization coefficient. Consistently, double-knockdown of Cdc42a/c, inhibition of actin polymerization by Latrunculin B treatment and suppression of Cdc42-dependent filopodia formation by Irsp53 4 K led to reductions of the signalling range ( Fig. 4h ). Similarly, the Mander’s co-localization was reduced by the knockdown, the inhibitor of actin polymerization and the expression of the IRSp53 4 K mutant ( Fig. 4i ). Next, we quantified the fluorescence intensity of cell nuclei of the 7xTCF-XLa.Siam:mCherry-NLS after introduction of a Wnt8a-positive clone ( Fig. 4j , Supplementary Fig. 4d ). We found that co-activation of Cdc42 in the Wnt8a-secreting clones led to an increase of the median intensity of the measured cell nuclei over basic activation, whereas knockdown of Cdc42, treatment with Latrunculin B or blockage of IRSp53 function led to reduced expression of the Wnt reporter in the host cells ( Fig. 4k ). Taken together, we conclude that Wnt8a-positive filopodia formation is strictly dependent on Cdc42 function and that these filopodia increase the effective Wnt signalling range in neighbouring cells ( Fig. 4l ). These data suggest a unique carrier and activation function for filopodia. Wnt filopodia extend primarily along the Wnt gradient Next, we tested whether such transport of signalling molecules has been proposed to promote the morphogenetic activity of Wnt proteins in larger tissues during vertebrate development. Wnt/β-catenin ligands are expressed at the margin of the posterior neural plate in vertebrates, and it has been proposed that graded Wnt activity is required for patterning the anteroposterior axis of the forebrain, midbrain and hindbrain [23] , [45] , [46] . According to this model, the Wnt source at the margin controls the fate of cells within the neural plate, cells that are located several tens of micrometres away from the cells producing the signalling molecule. To analyse the dynamics of Wnt distribution in early embryogenesis, we generated clones of ~10–15 cells that expressed fluorescently tagged Wnt8a in the presumptive neural plate ( Fig. 5a ). At the 50% epiboly stage, we segmented the receiving tissue of ~15 clones into 5 μm 3 cubes and measured the total fluorescence signal within each cube. We observed a halo of fluorescence at a distance of 10–20 μm away from the clone (arrows). We found 41.0±7.0% of the detected total fluorescence of the receiving tissue within this belt. Next, we quantified the directionality as well as the length of the filopodia of Wnt8a-expressing marginal cells (examined for 15 cells, Supplementary Fig. 2a ). We found that cells located in the marginal zone extended long filopodia, with a bias towards the animal pole of the embryo ( Fig. 5b ). In addition, we found that filopodia pointing towards the animal sector appear longer than control filopodia ( Fig. 5c ). These results suggest that cells producing Wnt8a at the margin extend specialized filopodia into the Wnt signalling field. Remarkably, the width of the detected belt of fluorescence around a Wnt8a clone corresponds to the average length of the measured filopodia, as 49.8% of filopodia pointing to the animal pole project into an area of 10–20 μm from the source ( Fig. 2d ). 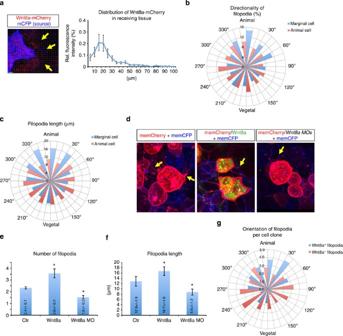Figure 5: Directed, filopodia-based transport of Wnt8a accounts for gradient formation. (a) Distribution of fluorescently tagged Wnt8a around a representative clone secreting Wnt8a-mCherry in the zebrafish neural plate at 50% epiboly. The highest fluorescence was detected in a halo around the clone (arrows). Quantification of total fluorescence in cubes of 5 μm3of receiving tissue; approximately 15 individual clones are displayed based on the distance from the source. (b) Using 15 isolated marginal cells, the directionality of filopodia (n=153) was compared with the directionality of filopodia from cells at the animal pole (n=96) and displayed in a wind rose plot. Here, 36.7% of filopodia analysed are directed towards the animal pole within a sector of ±30° (from 330° to 30°) compared with 23.2% that are directed towards the margin (150° to 210°). (c) Lengths of the same filopodia were measured, and the average lengths per segment were plotted according to their orientation. Filopodia directed towards the animal pole displayed an average length of 16.6±3.5 μm. Filopodia in the vegetal sector had an average length of 9.4±2.4 μm. Cells located at the animal pole had a random directionality distribution of 9.0±0.4% per segment and an average length of 11.7±1.8 μm of cell extensions. (d) Representativein vivoimage of 15-μm stacks of Cherry-GPI-positive cells injected with 0.2 ng Wnt8a-GFP mRNA or 4 ng Wnt8a Morpholino oligomeres in the mCFP-positive neural plate in zebrafish. Arrows mark Wnt8a-positive filopodia. (e) Number of filopodia of 15 individual cells was quantified from (d). (f) Quantification of the lengths of the filopodia from (e). (g) Quantification of Wnt8a-positive filopodia according to their projection direction in the embryo. In the wind rose plot, 0° represents the animal pole, and 180° the vegetal pole. Error bars represent the s.e.m. Significance level as indicated: *P<0.05. Figure 5: Directed, filopodia-based transport of Wnt8a accounts for gradient formation. ( a ) Distribution of fluorescently tagged Wnt8a around a representative clone secreting Wnt8a-mCherry in the zebrafish neural plate at 50% epiboly. The highest fluorescence was detected in a halo around the clone (arrows). Quantification of total fluorescence in cubes of 5 μm 3 of receiving tissue; approximately 15 individual clones are displayed based on the distance from the source. ( b ) Using 15 isolated marginal cells, the directionality of filopodia ( n =153) was compared with the directionality of filopodia from cells at the animal pole ( n =96) and displayed in a wind rose plot. Here, 36.7% of filopodia analysed are directed towards the animal pole within a sector of ±30° (from 330° to 30°) compared with 23.2% that are directed towards the margin (150° to 210°). ( c ) Lengths of the same filopodia were measured, and the average lengths per segment were plotted according to their orientation. Filopodia directed towards the animal pole displayed an average length of 16.6±3.5 μm. Filopodia in the vegetal sector had an average length of 9.4±2.4 μm. Cells located at the animal pole had a random directionality distribution of 9.0±0.4% per segment and an average length of 11.7±1.8 μm of cell extensions. ( d ) Representative in vivo image of 15-μm stacks of Cherry-GPI-positive cells injected with 0.2 ng Wnt8a-GFP mRNA or 4 ng Wnt8a Morpholino oligomeres in the mCFP-positive neural plate in zebrafish. Arrows mark Wnt8a-positive filopodia. ( e ) Number of filopodia of 15 individual cells was quantified from ( d ). ( f ) Quantification of the lengths of the filopodia from ( e ). ( g ) Quantification of Wnt8a-positive filopodia according to their projection direction in the embryo. In the wind rose plot, 0° represents the animal pole, and 180° the vegetal pole. Error bars represent the s.e.m. Significance level as indicated: * P <0.05. Full size image The formation of filopodia can be initiated in response to ligands such as FGF [47] . On the basis of the co-localization of Toca-1 with Wnt8a at filopodia nucleation points, we suspected that Wnt itself could play a role in the formation of filopodia, particularly because Wnt8a signal could be observed at the plasma membrane before the initiation of filopodia extension ( Supplementary Fig. 1f , Supplementary Movie 2 ). Indeed, we found increases in the number and length of filopodia in cells overexpressing Wnt compared with control cells ( Fig. 5d–f ). However, Wnt8a does not regulate the expression of Cdc42 ( Supplementary Fig. 5b ). Consistently, knockdown of Wnt8a reduced the number and length of the filopodia ( Fig. 5d–f ). We observed both Wnt8a-GFP-positive and -negative filopodia. To determine the reason behind observing both filopodia types, we correlated the direction of the filopodia with their Wnt8a content. We found that filopodia pointing towards the animal pole carry Wnt8a significantly more often than filopodia pointing towards the vegetal pole ( Fig. 5g ), suggesting that Wnt8a is preferentially transported along its gradient. Length of signalling filopodia influences tissue patterning Next, we investigated the effect of altered filopodia length on Wnt8a signalling activity and signalling range during early gastrulation stages. To this end, we first quantified Wnt activity in the embryo at 50% epiboly by analysing the relative expression levels of the target genes axin2 and lef1 by qRT-PCR. We found that the expression levels of both target genes were not significantly changed when filopodia length was altered by Cdc42 overexpression, Cdc42 knockdown, Latrunculin B treatment or overexpression of the IRSp53 4 K mutant ( Fig. 6a ). In addition, we found that the expression of the Wnt ligand is similarly unchanged under these conditions ( Fig. 6b ). However, we found significant increases in the expression of target genes after Wnt8a overexpression, which could be further increased by the co-expression of Cdc42 ( Fig. 6a ). 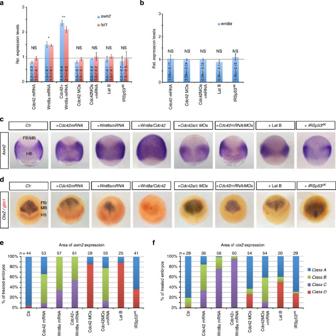Figure 6: Cdc42 dependent filopodia regulate gene expression in the neural plate. (a,b) Quantification of the expression levels of target genes and ligand by qRT-PCR. At the one-cell stage, embryos were injected with indicated constructs: Cdc42 mRNA, 0.6 ng; Wnt8a mRNA, 0.2 ng, IRSp534 KmRNA, 1.2 ng; Morpholino oligomers targeting Cdc42a and Cdc42c 4 ng each. Alternatively, embryos were treated with 25 nM Latrunculin B from 30% epiboly until 50% epiboly. Total mRNA was isolated from 50 embryos at 50% epiboly. Experiments were conducted in triplicates. (a) Relativeaxin2 and lef1expression levels and (b)wnt8aexpression levels are displayed relative to those in wild-type embryos (set to 1.0). Error bars, s.e.m. Significance levels as indicated: *P<0.05; **P<0.01. (c,d) Embryos at 75% epiboly were fixed and subjected toin situhybridization againstaxin2andotx2/gbx1. FB/MB, forebrain-midbrain anlage, HB, hindbrain anlage. (e,f) Embryos were sorted according to their phenotype into four classes (for details seeSupplementary Fig. 6a). (e) classification of embryos from (c): overexpression of 0.6 ng of Cdc42 mRNA (Class A:18; Class C:30; Class D:5); overexpression of 0.2 ng of Wnt8a mRNA (C:37; D:20); co-expression of Cdc42 and Wnt8a mRNA (C:28; D:33); knockdown of Cdc42a/c (A:4; B:24), rescue of knockdown by co-expression of Cdc42 mRNA (A:13; C:38; D:8); treatment with Latrunculin B (A:3; B:22) and overexpression of 1.2 ng of IRSp534 K(A:2, B:50). (f) classification of embryos from (d): Overexpression of Cdc42 (A:6; B:19; C:11); Wnt8a (A:1; B:15; C:42); co-expression of Cdc42 and Wnt8a (B:3; C:57); knockdown of Cdc42a/c (A:34; B:6; C14), rescue of knockdown by co-expression of Cdc42 mRNA (A:14; B:16; C:4); Latrunculin B treatment (A:8; B:2; D:10) and overexpression of IRSp534 K(A:2, D:50). Figure 6: Cdc42 dependent filopodia regulate gene expression in the neural plate. ( a , b ) Quantification of the expression levels of target genes and ligand by qRT-PCR. At the one-cell stage, embryos were injected with indicated constructs: Cdc42 mRNA, 0.6 ng; Wnt8a mRNA, 0.2 ng, IRSp53 4 K mRNA, 1.2 ng; Morpholino oligomers targeting Cdc42a and Cdc42c 4 ng each. Alternatively, embryos were treated with 25 nM Latrunculin B from 30% epiboly until 50% epiboly. Total mRNA was isolated from 50 embryos at 50% epiboly. Experiments were conducted in triplicates. ( a ) Relative axin2 and lef1 expression levels and ( b ) wnt8a expression levels are displayed relative to those in wild-type embryos (set to 1.0). Error bars, s.e.m. Significance levels as indicated: * P <0.05; ** P <0.01. ( c , d ) Embryos at 75% epiboly were fixed and subjected to in situ hybridization against axin2 and otx2/gbx1 . FB/MB, forebrain-midbrain anlage, HB, hindbrain anlage. ( e , f ) Embryos were sorted according to their phenotype into four classes (for details see Supplementary Fig. 6a ). ( e ) classification of embryos from ( c ): overexpression of 0.6 ng of Cdc42 mRNA (Class A:18; Class C:30; Class D:5); overexpression of 0.2 ng of Wnt8a mRNA (C:37; D:20); co-expression of Cdc42 and Wnt8a mRNA (C:28; D:33); knockdown of Cdc42a/c (A:4; B:24), rescue of knockdown by co-expression of Cdc42 mRNA (A:13; C:38; D:8); treatment with Latrunculin B (A:3; B:22) and overexpression of 1.2 ng of IRSp53 4 K (A:2, B:50). ( f ) classification of embryos from ( d ): Overexpression of Cdc42 (A:6; B:19; C:11); Wnt8a (A:1; B:15; C:42); co-expression of Cdc42 and Wnt8a (B:3; C:57); knockdown of Cdc42a/c (A:34; B:6; C14), rescue of knockdown by co-expression of Cdc42 mRNA (A:14; B:16; C:4); Latrunculin B treatment (A:8; B:2; D:10) and overexpression of IRSp53 4 K (A:2, D:50). Full size image Next, we analysed the distribution of axin2 transcripts within the embryo, sorting them according to their expression pattern into four phenotypic classes: normal (class A), expanded (class B), severely expanded (class C) and reduced (class D; Supplementary Fig. 5a ). Increasing the filopodia length by overexpression of Cdc42 resulted in an expansion of the axin2 expression domain as manifested by an increase in class B embryos ( Fig. 6c,e ). Similar expansion was detected on expression of Wnt8a mRNA. Co-expression of Cdc42 and Wnt8a mRNA led to a synergistic effect and significant enhancement of class C embryos. Knockdown of Cdc42 led to a reduced axin2 expression area and an enhanced number of class D embryos, which could be rescued by co-expression of Cdc42 mRNA. Inhibiting the formation of filopodia by treatment with Latrunculin B or overexpression of IRSp53 4 K also led to a reduced area of axin2 expression ( Fig. 6c,e ). In summary, we found that the levels of the ligand and target gene production were not altered by filopodia formation. The range of Wnt/β-catenin signalling, however, was correlated with the length and number of functional filopodia. Inhibiting or enhancing the formation of filopodia thus led to a shorter signalling range with a steeper signal gradient or to a longer signalling range with a shallower slope of Wnt distribution, respectively. Next, we analysed the expression of the neural patterning gene otx2 , a marker of the forebrain and the midbrain anlage in the neural plate at early gastrulation stages ( Fig. 6d ) that is directly suppressed by Wnt/β-catenin [23] . On the basis of the expression pattern, we grouped the embryos into four categories: A, normal; B, reduced; C, severely reduced; D, expanded ( Supplementary Fig. 5a ). We found that the expression of otx2 was reduced after the overexpression of Cdc42 or Wnt8a, thereby increasing the numbers of embryos displaying the class B and class C phenotypes. Furthermore, we observed a synergistic effect when the two mRNAs were combined. Functional blockage of Cdc42a/c led to an expansion of the otx2 expression domain that could be rescued by co-expression of Cdc42 mRNA in double-morphant embryos. Latrunculin B treatment or overexpression of IRSp53 4 K led to an expansion of otx2 expression. Blockage of Cdc42 or inhibition of actin polymerization may lead to alterations in cell migratory events such as epiboly, gastrulation and convergent extension at the same time [48] . Here, we found that patterning within the neural plate was altered. Together, our results are consistent with the notion that alterations in the properties of the filopodia affect the distribution of Wnt8a, thereby altering the patterning of the neural plate. Simulation of Wnt distribution in the neural plate To examine our hypothesis quantitatively, we developed a simulation of neural plate patterning ( Fig. 7a ; Supplementary Fig. 5a ). The simulation takes into account ligand transport by filopodia, ligand decay and the migration of epiblast cells using a Monte-Carlo simulation approach [49] and is based on measured experimental parameters, such as filopodia angle and length distribution (see Supplementary Fig. 5b for further details). Employing filopodia as the exclusive transport mechanism from the producing layer to the epiblast layer and cell intermingling, we found that Wnt8a can be distributed in a graded manner over the entire neural plate ( Fig. 7a , Supplementary Movie 6 ). Furthermore, we found that the simulated concentration of the ligand peaked at 50 μm from the body of the producing cells, forming a corona around the source tissue, consistent with our previous observations of Wnt8a-mCherry distribution ( Fig. 5a ). Next, we tested three scenarios with varying filopodia lengths and frequencies, based on our clonal in vivo measurements ( Fig. 4e ). We found that ligand concentration within the entire morphogenetic field depends on the length of the filopodia. Indeed, we observed low contact frequencies with the epiblast cells resulting in lower Wnt8a concentrations for lower filopodia lengths. If we required that all filopodia hit a target cell in the epiblast cell layer with a 100% success rate, there were only minimal differences in the concentration of the ligand within the morphogenetic field for different filopodia lengths ( Supplementary Fig. 6e ) because different filopodia lengths simply shift the gradient by the length difference. Remarkably, we found that increasing the length of the filopodia led to a wider distribution (shift on the x-axis), whereas an increase in the frequency of filopodia formation increased the ejection of the ligand and primarily affected the nearest neighbouring cells (shift on the y-axis) and only subsequently affected the range of the distribution. 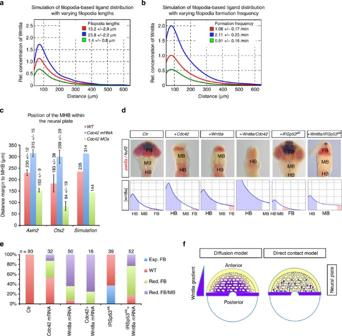Figure 7: Simulation and experimental validation of Wnt transport on CNS patterning. (a,b) A Monte-Carlo based simulation (detailed parameters listed inSupplementary Fig. 5) was generated, and it displayed the hypothetical distribution of a ligand such as Wnt8a from source cells with indicated filopodia lengths and formation frequency in a morphogenetic field of 600 μm after 3.4 h of development (Supplementary Movie 6). For the neural plate, we used a box of size 5,000 × 1,000 μm2with 17,490 discrete cell positions and a cell diameter of 16 μm. The simulation started at 4.6 hpf (30% epiboly), when Wnt8a expression is first detected. The Wnt8a-positive marginal zone was set to a 40-μm broad layer containing 650 ligand-producing cells and the receiving tissue—the neural plate anlage—was set to a 50-μm broad layer containing 888 epiblast cells. At 8 hpf (75% epiboly stage), the simulation was stopped when the neural plate was extended to 600 μm and anteroposterior patterning could be determined by marker gene expression. During the simulation, the producing marginal cell population was kept constant. (c) The position of the midbrain-hindbrain boundary (MHB) was measured in 15 representative embryos from wt, Cdc42 mRNA-injected and Cdc42-knockdown groups inFig. 6c,d, and the distance from the margin to the MHB is displayed. These data were compared with values calculated from the simulation. (d) Embryos were microinjected with mRNA for the indicated constructs (Cdc42, 0.6 ng; Wnt8a, 0.2 ng; IRSp534 K, 1.2 ng) at the one-cell stage. Embryos were fixed at 26 hpf and subjected toin situhybridization with probes forfezf2andpax6a. (e) Embryos were classified according to the presence of the three anlagen of major brain parts: FB, forebrain; MB, midbrain; and HB, hindbrain. (f) Comparison of the established morphogen diffusion model to the filopodia-based direct contact model (explanation in text). Figure 7: Simulation and experimental validation of Wnt transport on CNS patterning. ( a , b ) A Monte-Carlo based simulation (detailed parameters listed in Supplementary Fig. 5 ) was generated, and it displayed the hypothetical distribution of a ligand such as Wnt8a from source cells with indicated filopodia lengths and formation frequency in a morphogenetic field of 600 μm after 3.4 h of development ( Supplementary Movie 6 ). For the neural plate, we used a box of size 5,000 × 1,000 μm 2 with 17,490 discrete cell positions and a cell diameter of 16 μm. The simulation started at 4.6 hpf (30% epiboly), when Wnt8a expression is first detected. The Wnt8a-positive marginal zone was set to a 40-μm broad layer containing 650 ligand-producing cells and the receiving tissue—the neural plate anlage—was set to a 50-μm broad layer containing 888 epiblast cells. At 8 hpf (75% epiboly stage), the simulation was stopped when the neural plate was extended to 600 μm and anteroposterior patterning could be determined by marker gene expression. During the simulation, the producing marginal cell population was kept constant. ( c ) The position of the midbrain-hindbrain boundary (MHB) was measured in 15 representative embryos from wt, Cdc42 mRNA-injected and Cdc42-knockdown groups in Fig. 6c,d , and the distance from the margin to the MHB is displayed. These data were compared with values calculated from the simulation. ( d ) Embryos were microinjected with mRNA for the indicated constructs (Cdc42, 0.6 ng; Wnt8a, 0.2 ng; IRSp53 4 K , 1.2 ng) at the one-cell stage. Embryos were fixed at 26 hpf and subjected to in situ hybridization with probes for fezf2 and pax6a . ( e ) Embryos were classified according to the presence of the three anlagen of major brain parts: FB, forebrain; MB, midbrain; and HB, hindbrain. ( f ) Comparison of the established morphogen diffusion model to the filopodia-based direct contact model (explanation in text). Full size image On the basis of the expression analysis of neural plate markers ( Fig. 6b,c ) and on the simulation ( Fig. 7a ), we hypothesized that filopodia length and formation frequency should affect the distribution of the ligand and hence on the anteroposterior patterning of the neural plate. To analyse the effect of altered filopodia length on ligand distribution, we measured the position of a landmark that is easy to identify experimentally, the midbrain-hindbrain boundary (MHB; Fig. 7b ). To determine the position of the MHB within the neural plate, we measured the distance of the axin2 expression from the margin to the anterior limit of the expression domain ( Fig. 6c ), which specifies the position of the MHB. When Cdc42 was activated, we found that the axin2 expression border at the MHB was shifted anteriorly by 27%. Consistently, we found a 33% posterior shift of the axin2 expression border at the MHB in embryos with inhibited Cdc42a/c function. These observations could be verified by quantifying the position of the MHB based on expression of the forebrain/midbrain marker otx2 ( Fig. 6d ), which was determined by the distance of the anterior neural border of the neural plate to the posterior border of the otx2 expression domain and subtracted from the length of the entire neural plate. The position of the WT MHB was observed to shift anteriorly by 39% when Cdc42 was overexpressed and posteriorly by 53% when Cdc42 function was inhibited. To verify the simulation from Fig. 7a , we next analysed the effect of Cdc42-mediated filopodia formation on early neural plate patterning. On the basis of the experimentally measured position of the MHB in WT embryos, we calculated the relative position of the MHB in the simulation when the filopodia length and formation frequency were increased or decreased. Remarkably, we found a similar scenario in our mathematical simulation: a 25% anterior shift of the position of the MHB when the filopodia length was increased and a 39% posterior shift when the filopodia length was decreased ( Fig. 7b ). This result validated our simulation model, and it suggests that filopodia length is an important parameter for determining ligand concentration within the entire morphogenetic field and that Wnt transport on filopodia provides an important mechanism for anteroposterior patterning in the neural plate. If Cdc42 facilitates the distribution of Wnt signals in early embryogenesis, we would expect severe consequences on the development of the central nervous system at later embryonic stages. To test this hypothesis, we marked the primordia of the anterior forebrain with fezf2 and the anlage of the posterior forebrain and the hindbrain with pax6a [50] ( Fig. 7d ). Overexpression of Cdc42 mRNA led to a reduction in the size of the fezf2 -positive presumptive anterior forebrain compared with control embryos, suggesting that Cdc42-mediated formation of the filopodia facilitates Wnt/β-catenin signalling during neural plate patterning. Indeed, a similar reduction in the size of anterior brain structures was observed in embryos injected with a low dose of Wnt8a mRNA (0.2 ng), and co-expression of Cdc42 and Wnt8 produced a synergistic anterior truncation of the neural tube and the absence of the pax6a -positive forebrain and the pax6a -negative midbrain. Next, we blocked the formation of filopodia by overexpressing an Irsp53 4 K mutant. We found that the embryos displayed posterior expansion of the anterior brain structures and that the fezf2 and pax6 expression domains were expanded in these embryos ( Fig. 7d,e ), similar to a phenotype displayed when Wnt antagonists, such as dickkopf-1, are activated. By providing a low concentration of Wnt8a mRNA, the phenotype of the IRSp53 4 K mutant could be rescued ( Fig. 7d,e ), suggesting that the filopodia play a major role in distributing Wnt ligands in early development. In summary, we conclude that the transport of Wnt/β-catenin on filopodia is important for establishing positional information in the developing central nervous system. Cell–cell communication by signalling proteins is fundamental for the regulation of differentiation and growth. Understanding the mechanisms responsible for the transport and distribution of signalling proteins is therefore important for the understanding of tissue patterning events and embryonic development. Transport of signalling molecules can occur by free diffusion [24] or planar transcytosis [51] or on exovesicles, such as argosomes [52] , lipoproteins [53] or exosomes [8] , [10] . In these mechanisms, the formation of a gradient is based on parameters such as the ligand concentration in the extracellular matrix (ECM), the interaction between the ligand and the ECM (sticky versus non-sticky) and the diffusion rate of the ligand ( Fig. 7f ). According to an alternative model, signalling molecules are delivered directly to the receiving cells via specialized cell protrusions termed cytonemes [11] . In such a direct-contact model, parameters such as cytoneme length, the speed of cytoneme formation, ligand concentrations on these extensions and the contact frequency of the target cell dictate the properties of the morphogenetic gradient. In this study, we provide evidence that the paracrine transport of canonical Wnt8a during zebrafish neural plate patterning is facilitated by specialized filopodia ( Fig. 7f ). Are Wnt-transporting filopodia cytonemes? In recent years, evidence for the transport of signalling proteins such as Hh [15] or Dpp [54] on cytonemes has increased, and ligand-producing cells have been suggested to form cytonemes to contact responding cells over a distance [55] . In the classic view, cytonemes are thought to contact ligand producing cells, and these fragile structures are not preserved during conventional fixation. In contrast, the Wnt-positive filopodia that we describe in zebrafish are relatively short, extending only a few tens of micrometres. These filopodia present the ligand at their tips and contain fixable, Cdc42-dependent parallel actin bundles. However, recently a revised definition of the cytoneme model places no distinction on length or on the distribution of ligand within or on them [14] , [55] . Therefore, we suggest that in the context of early patterning of the neural plate, Wnt is distributed by short protrusions, which may fit to the novel definition of cytonemes as signalling filopodia. Are there additional distribution mechanisms operating in parallel to filopodia during neural plate patterning? Although the expression level of the ligand was unaltered in our experiment ( Fig. 6b ), inhibition of filopodia formation markedly reduced the signalling range ( Fig. 4g ). In parallel, we were unable to find more Wnt8a in the supernatant after changes in Cdc42 function ( Fig. 4c ). Although we cannot exclude the possibility that other mechanisms contribute to the distribution of Wnt to a certain degree, the effects of manipulating filopodia formation on ligand distribution and on the patterning of the brain anlage suggest a critical role for the transport of Wnt ligand via filopodia during early gastrulation. Recent data from Drosophila may support our hypothesis: a membrane-tethered form of Wg was able to substitute for WT-Wg without major consequences during Drosophila wing development [5] . Although Wg-positive filopodia were not observed in this study [5] , such mechanism would allow the controlled dispersal of Wnt/Wg in a tissue without the need for free diffusion. We further hypothesize that the establishment of the Wnt gradient by filopodia could be achieved by differences in ligand concentration carried by filopodia or by differences in the contact frequency. Control of ligand concentration on filopodia has thus far not been shown; however, a mechanism based on contact frequency based has recently been suggested for Hh gradient formation [56] . How can Wnt generate a long-range signalling gradient in vertebrates? The ‘gradient by inheritance’ mechanism is one possible explanation for this phenomenon. Here, the gradients for the distribution of posterior morphogens such as Wnt3a along the mouse and chick embryonic axes are established by the decay of mRNA or protein in a cell flow [57] . A different mechanism for neural crest development has recently been suggested. Here, Wnt-producing cells can distribute the ligand by active cell migration over long distances [58] . In both of these models, the ligand-producing cells leave the signalling zone and contribute to the responding tissue. However, during formation of the neural plate, the neural ectoderm does not express Wnt8a [59] . The only ligand-producing cells are the Brachyury/Ntl-positive mesendodermal progenitors at the margin [60] , and tracking of all cells during zebrafish gastrulation showed that the marginal mesendoderm progenitors are strictly separated from the anterior-located neural ectoderm [61] . The same authors showed that the elongation of the neural plate in anteroposterior direction during gastrulation results from a mix of epiboly movement and an orthogonal intercalation of neural ectodermal cells ( Supplementary Fig. 5a ). We hypothesize that at the initiation of Wnt8a expression at 4 hpf, all neural ectodermal cells are within reach of the Wnt-positive filopodia from the Wnt8a-positive marginal cells. Our hypothesis implies that these contacted cells retain Wnt activity for the next several hours during neural plate patterning. Activation of the Wnt signalling cascade, including translocation of signal-mediating β-catenin into the nucleus and subsequent expression of target genes such as Axin2, has already begun after 30 min. However, analysis of the dynamics of the Wnt transduction cascade showed that the maximal activation plateau was not reached until 2 h of Wnt stimulation [62] . The signalling cascade might then be resolved again by the activation of the β-catenin destruction complex through GSK3-mediated phosphorylation of Axin1 [63] . The activation and deactivation dynamics of this process would therefore fit with a prolonged signalling activity in cells until 8 hpf (75% epiboly), when the Wnt-mediated patterning of the neural plate is set. Indeed, we found that the width of the expression area of the direct target gene axin2 continuously broadened within the neural plate between 4 hpf and 8 hpf (compare Supplementary Fig. 5b and Fig. 6c ). It seems that formation of signalling filopodia in vertebrates is a complex process and does not follow a unique regime. We show that Wnt8a is transported on Cdc42-dependent filopodia, whereas recent data suggest that Shh-positive filopodia in chick uses an Cdc42-independent mechanism [16] . It will be interesting to decipher whether certain types of filopodia are required for the propagation of specific ligands. Furthermore, it has been suggested that contacting of filopodia to a certain substratum may hinder filament assembly, thereby leading to changes that promote retraction and collapse [64] . Indeed, we found that the outgrowth of Wnt-positive filopodia did not guarantee the dispersal of the ligand. In many cases, we observed that the cells retracted the filopodia with Wnt8a, and we assume that this is because the correct target cell was not found. This observation became relevant for the generation of the morphogenetic field in our simulation. When the simulation required that all filopodia deliver the ligand to any neighbouring cells with a full success rate, we observed only minimal differences in the concentration of the ligand within the morphogenetic field, although the filopodia lengths were doubled ( Supplementary Fig. 5e ). We concluded that for generating a gradient employing the mechanism we describe, it is essential to retract the filopodium if the correct target cell is not in reach, instead of delivering the factor to a random next-door neighbour. The net change in the flux of Wnt8a from producing to receiving tissue controls the range of the gradient and is directly proportional to the filopodia length. We suggest that a filopodia-based distribution mechanism for Wnt8a is essential for patterning the neural plate during early zebrafish development. In addition, our experiments with various vertebrate cell lines suggest that this might be a general mechanism independent of early developmental processes, and it will be interesting to investigate in which contexts a filopodia-based propagation mechanism for Wnts is also important. Cell culture experiments Experiments were performed in zebrafish PAC2 fibroblasts derived from 24 h old embryos and maintained in Lebowitz-15 media and supplemented with 15% fetal bovine serum ad 5% embryo extract, generously provided by in Nicholas Foulkes (KIT). Human HEK293T cells (Embryonic kidney cells; CRL-1573) and mouse NIH/3T3 cell line (mouse embryonic fibroblast; CRL-1658) were both revceived from American tissue culture collection, ATTC, Wesel, Germany. All the material used for cell culture was purchased from Life Technologies, Gibco. For transfection experiments FuGENE HD Transfection Reagent (Promega) or ScreenFect (InCella) was used. The Super TopFlash (STF) reporter gene assay uses the expression of the enzyme luciferase driven by a 7xTcf responsive element [40] to measure Wnt signalling activity. The luciferase activity was monitored using the in vivo luminometer (Envision, Perkin Elmer). Primary cell cultures were derived from blastula embryo by explanting cell from the marginal and the animal pole to a petri dish; the explant procedure has been performed with a standard transplantation set-up; the cells were then cultivated for 24 h in Leibovitz’s L-15 medium with 15% FBS, 1% Pen/Strep and 0.1% Gentamicin at 28 °C and without additional CO 2 supply, similar to PAC2 fibroblast. Activity of the supernatant was analysed in the following way. Supernatant of transfected HEK293T cells with empty plasmid, Wnt8a, Wnt8a+Cdc42 WT , Wnt8a+Cdc42 T17N , Wnt8a+IRSp53 4 K or cells transfected with Wnt8a and treated with Latrunculin B were filtered through a 0.22-μm filter. After 1 h of exposure of HEK293T cells transfected with a STF reporter to the supernatant, the reporter activity was monitored for 6 h. All cell culture experiments were carried out in triplicates. Fish embryo experiments All zebrafish husbandry and experimental procedures were performed in accordance with the German law on Animal Protection and were approved by Local Animal-Protection Committee (Regierungspräsidium Karlsruhe, Az.35-9185.64) and the Karlsruhe Institute of Technology (KIT). Breeding zebrafish ( Danio rerio ) were maintained at 28 °C on a 14 h light/10 h dark cycle. To prevent pigment formation, embryos were raised in 0.2 mM 1-phenyl-2-thiourea (PTU, Sigma, St Louis, MO 63103 USA) after 24 hpf. The data we present in this study were acquired from analysis of KIT wild-type zebrafish AB 2 O 2 and Tg(7xTCF-XLa.Siam:mCherry-NLS) ia4 [51] . Plasmids and Morpholino oligomers Transient knockdown of gene expression was performed by a Morpholino-antisense oligomere approach. The following antisense oligomers (MO) were used: Cdc42a MO 5′- AACGACGCACTTGATCGTCTGCATA -3′; Cdc42c MO 5′- CACCACACACTTTATGGTCTGCATC -3′; and Wnt8a MOs [65] . The used concentration per Morpholino oligomer was 5 nmol μl −1 and microinjected at the one-blastomere stage into the yolk. For the overexpression studies the following plasmids have been used: zfWnt8 ORF1-GFP in pCS2+ [23] , zfWnt8 ORF1-mCherry in pCS2+, pcDNA3-EGFP-Cdc42 WT [41] ; Addgene 12975), pcDNA3-EGFP-Cdc42 T17N (Addgene 12976), Dvl2-mcherry in pCS2+, pCMV-hEvi-Cherry [8] , Super8xTopFlash in pTA-Luc. [40] , pmKate2-f-mem (Evrogen), GPI-anchored mCherry in pCS2+, LRP6-GFP in pCS2+ [66] , DCK-GFP [32] , N-WASP-GFP [33] (Addgene 33019), GFP-wGBD [67] (Addgene 26734), EGFPC1-MyoX [68] (Addgene 47608), IRSp53-GFP and IRSp53 4 K [37] . The following antisense RNA probes have been used: axin2 , otx2 ; pax6a and fezf2 [69] . For the immunostaining of Wnt-producing cells, a polyclonal Wnt8a antibody (1:100, No. 9735; One World Lab), Alexa Fluor 488 Goat Anti-Rabbit secondary antibody (1:1,000, No. A11008; Life Technologies), phalloidin (P1951, Sigma) and DAPI (D9542, Sigma) were used. Cells were fixed at RT for 20 min in PFA 4%, washed in PBS and permeabilized with 0.05% TritonX-100 solution in PBS for 15 min. To block unspecific binding of antibodies, cells were incubated with 1% BSA in PBS o/n at 4 °C. The primary antibody was added and diluted in 3%BSA/PBS for 2 h at RT. Cells were washed in PBS and incubated with the secondary antibody for 60 min at RT. Finally, cells were washed and incubated with 50 μg ml −1 phalloidin and for 40 min and 10 μg μl −1 DAPI for 5 min at RT. Experimental procedures For the chemical treatment, cell cultures were treated with Cytochalasin D 5 μM (Enzo Life Science) Latrunculin 25 nM (Enzo Life Science), Cdc42/Rac1 GTPase Inhibitor, ML141 10 μM (Merck Millipore) for 2 h and analysed. Zebrafish embryos were treated with 0.25 nM Latrunculin B (1%DMSO v/v) from 30 to 70% epiboly stages. The injection of mRNAs and Morpholino oligomers was performed according to the description in the text. Capped and in vitro transcribed mRNA, (mMessage Machine Kit, Ambion) was microinjected into one of 16 cells to generate cell clones [36] . Embryos were incubated at 28 °C at shield stage and fixed for whole-mount mRNA in situ hybridization (ISH) or subjected to microscopical analysis at indicated stages. For real-time quantitative PCR (qRT-PCR), 50 embryos each were lysed in 300 μl TriZol (Sigma), and total RNA was prepared using Direct-zol RNA Mini Prep Kit from Zymo Research. cDNA was prepared using MMLV reverse transcriptase from Promega and analysed in a Real-Time PCR system from LifeTechnologies (ABI StepOnePlus). Primers with the following sequence were used: beta-Actin (Forward: 5′- CCTTCCTTCCTGGGTATGG -3′; Reverse: 5′- GGTCCTTACGGATGTCCAC -3′), Axin2 (Forward: 5′- CAATGGACGAAAGGAAAGATCC -3′; Reverse: 5′- AGAAGTACGTGACTACCGTC -3′), Lef1 (Forward: 5′- CAGACATTCCCAATTTCTATCC -3′; Reverse: 5′- TGTGATGTGAGAACCAACC -3′), Cdc42 (Forward: 5′- AACCCATCACTCCAGAGAC -3′; Reverse: 5′- CATTCTTCAGACCTCGCTG -3′) and Wnt8a (Forward: 5′- CTATATGCTGTCACATACTGTCG -3′; Reverse: 5′- ATGCGAGATAAGCCTTTGGT -3′). For in-situ hybridization, digoxygenin- and fluorescein-labelled probes were prepared from linearized templates using an RNA labelling and detection kit (Roche) [50] . Embryos were transferred to 70% Glycerol/PBS (v/v). Images were taken on an Olympus SZX16 microscope equipped with a DP71 digital camera by using Cell A imaging software. For confocal analysis, live embryos were embedded in 0.7% low melting Agarose (Sigma-Aldrich) dissolved in 1 × Ringer’s solution. Images were obtained with a Leica TCS SP5 X confocal laser-scanning microscope using × 63 dip-in objective. Image processing was performed with Imaris 7.1 software (Bitplane AG, Switzerland). All experiments were carried out at least in biological triplicates if not indicated otherwise. Error bars indicate s.e.m. For figure 3,4,5, and 6 statistical significance was calculated by carrying out Student’s t -test. Simulations Computer simulations have been implemented in python using the libraries numpy, scipy and matplotlib [70] . A complete list of simulation parameters is reported in Supplementary Fig. 5 . How to cite this article: Stanganello, E. et al . Filopodia-based Wnt transport during vertebrate tissue patterning. Nat. Commun. 6:5846 doi: 10.1038/ncomms6846 (2015).